Reduced IFNλ4 activity is associated with improved HCV clearance and reduced expression of interferon-stimulated genes Hepatitis C virus (HCV) infections are the major cause of chronic liver disease, cirrhosis and hepatocellular carcinoma worldwide. Both spontaneous and treatment-induced clearance of HCV depend on genetic variation within the interferon-lambda locus, but until now no clear causal relationship has been established. Here we demonstrate that an amino-acid substitution in the IFNλ4 protein changing a proline at position 70 to a serine (P70S) substantially alters its antiviral activity. Patients harbouring the impaired IFNλ4-S70 variant display lower interferon-stimulated gene (ISG) expression levels, better treatment response rates and better spontaneous clearance rates, compared with patients coding for the fully active IFNλ4-P70 variant. Altogether, these data provide evidence supporting a role for the active IFNλ4 protein as the driver of high hepatic ISG expression as well as the cause of poor HCV clearance. Hepatitis C virus (HCV) infections are the major cause of chronic liver disease, cirrhosis and hepatocellular carcinoma worldwide [1] . HCV is parenterally transmitted, mainly due to injection drug use, unsafe transfusions and therapeutic injections. In 70–80% of those infected, the virus persists and the infection becomes chronic, and eventually requires antiviral therapy. During the past 25 years, recombinant interferon-alpha (IFNα) has been an essential component of HCV treatment [2] , however, the recent availability of potent direct-acting antiviral agents (DAA) is changing the therapeutic options. The overall sustained virological response (SVR) rate achieved using a combination of pegylated IFNα (pegIFNα) and ribavirin is only about 50%, and the prognosis for individual patients strongly depends on their genetic background. In particular, the genetic variation within the IFNL3 (IL28B) locus is crucial in determining the treatment outcome [3] , [4] , [5] , [6] . Furthermore, the response to IFN-based therapy depends strongly on the expression of IFN-stimulated genes (ISGs) in patients before the initiation of treatment [7] , [8] , [9] and variations near the IFNL3 ( IL28B ) locus correlate with the ISG induction in the liver [10] , [11] , [12] . Somewhat paradoxically, patients showing increased pretreatment expression of ISG in the liver respond poorly to pegIFNα/ribavirin therapy [7] , [8] , [9] . However, the mechanism responsible for driving ISG induction in the HCV-infected liver has remained elusive. Roughly, a quarter of HCV-infected individuals clear the virus spontaneously, this largely happens during the acute phase of the infection. Somewhat surprisingly, the genetic variations near the IFNL3 ( IL28B ) locus are also strongly associated with spontaneous clearance of HCV infection [13] , [14] . That points towards a pivotal role for IFNλs in HCV clearance and a possible influence of IFNλs on the adaptive immune response that is generated during the acute phase of HCV infection. A recent key discovery identified the IFNL4 gene and showed that a polymorphism ( rs368234815 ), which causes the disruption of the IFNL4 reading frame, correlates with a substantially better treatment response [15] , [16] as well as better spontaneous clearance rate [13] . Thus, patients having a nonfunctional IFNL4 gene are more likely to clear the HCV infection. This suggests that the production of IFNλ4 in carriers of the ancestral rs368234815 ΔG allele is responsible for the transcriptional activation of ISGs, thus providing a molecular link between the genotype and clearance of HCV. This hypothesis is supported by the recent finding that recombinant IFNλ4 protein strongly stimulates Jak-STAT signalling and ISG induction through binding to the IFNλ receptor [17] . Here we describe a strong link between a reduced antiviral activity of the IFNλ4 protein and a reduced hepatic ISG expression as well as an improved HCV clearance. Substitution at position 70 impairs the activity of IFNλ4 Three non-synonymous single-nucleotide polymorphisms (SNPs) in the IFNL4 gene were previously described but not characterized [15] , [18] , those being C17Y ( rs73555604 ), R60P ( rs142981501 ) and P70S ( rs117648444) . We noted that a P70S substitution ( rs117648444 ) could potentially alter the activity of the protein, in addition this has a minor allele frequency (MAF) in Caucasian of 0.11 (HapMap), whereas the two other have 0 and 0.025, respectively. Proline 70 is located outside of the assumed receptor binding site [19] , [20] , but structural modelling suggests that P70 is important for the stability of the IFNλ4 protein [17] . In the following, the two variants of IFNλ4 will be denoted as IFNλ4-P70 and IFNλ4-S70, respectively. We expressed the mature form of both variants in Escherichia coli , purified them ( Fig. 1a ) and tested their activity. The IFNλ4-S70 variant induced significantly lower levels of both MX1 and IFIT1 transcription in human hepatocellular carcinoma cells (HepG2; Fig. 1b ). Next, a dose–response experiment was performed in human embryonic kidney cells (HEK293) transfected with an IFN-responsive firefly luciferase reporter construct, a Renilla luciferase construct for normalization and a construct expressing the IFNλR1 receptor chain ( Fig. 1c ). We obtained half-maximal effective concentration (EC 50 ) values of 4.0 ng ml −1 for IFNλ4-P70 and 9.5 ng ml −1 for IFNλ4-S70. 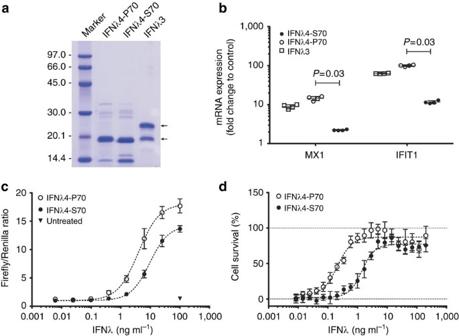Figure 1: Activity of recombinant human IFNλ4-P70 and IFNλ4-S70 variants. Data represent the results of multiple experiments with similar results. (a) A coomassie-stained 12% SDS–polyacrylamide gel electrophoresis of the purified proteins. Cleavage of the N-terminal His-Tag was only partial for IFNλ3, hence the double band. The upper arrow indicates the migration of the IFNλ3-His-tag fusion protein; the lower arrow indicates migration of the mature IFNλ3/λ4 proteins. (b) HepG2 cells were treated with 1 ng ml−1of IFNλ3, IFNλ4-P70 or IFNλ4-S70. After 4 h, the mRNA levels of the ISGsIFIT1andMX1were quantified by real-time quantitative PCR. Experiments were performed in quadruplicates; replicates, mean and s.d. are plotted. ThePvalue for IFNλ4-P70 versus IFNλ4-S70 is shown (Mann–Whitney test). (c) The activity of IFNλ4-S70 was tested and compared with IFNλ4-P70 in HEK293 cells, which were transfected with the pEF2 vector containing IFNλR1, as well asRenillaand firefly luciferase reporters 24 h before IFN treatment. The firefly construct is IFN inducible, whereas theRenillaconstruct is constitutively expressed. Dose responses of IFNs were performed in quadruplicates. Mean and s.d. are shown. (d) HepG2 cells were treated with IFNλ4-S70 or IFNλ4-P70 for 24 h and subsequently infected with EMCV. Cell survival was analysed using the conversion of MTT to formazan in living cells by measurement of theA600. Data are presented as a percentage of a non-infected cell control. Error bars depict s.d. of 10 replicates. This difference was significant using 99% confidence intervals ( Supplementary Table 1 ). Finally, we performed an antiviral assay using encephalomyocarditis virus (EMCV) infection in HepG2 cells ( Fig. 1d ; Supplementary Table 1 ). Here we saw a significant shift in the (EC 50 ) values from 0.2 ng ml −1 for the IFNλ4-P70 to 1.4 ng ml −1 for IFNλ4-S70. Thus, the IFNλ4-S70 variant is substantially less active than the IFNλ4-P70 variant. Figure 1: Activity of recombinant human IFNλ4-P70 and IFNλ4-S70 variants. Data represent the results of multiple experiments with similar results. ( a ) A coomassie-stained 12% SDS–polyacrylamide gel electrophoresis of the purified proteins. Cleavage of the N-terminal His-Tag was only partial for IFNλ3, hence the double band. The upper arrow indicates the migration of the IFNλ3-His-tag fusion protein; the lower arrow indicates migration of the mature IFNλ3/λ4 proteins. ( b ) HepG2 cells were treated with 1 ng ml −1 of IFNλ3, IFNλ4-P70 or IFNλ4-S70. After 4 h, the mRNA levels of the ISGs IFIT1 and MX1 were quantified by real-time quantitative PCR. Experiments were performed in quadruplicates; replicates, mean and s.d. are plotted. The P value for IFNλ4-P70 versus IFNλ4-S70 is shown (Mann–Whitney test). ( c ) The activity of IFNλ4-S70 was tested and compared with IFNλ4-P70 in HEK293 cells, which were transfected with the pEF2 vector containing IFNλR1, as well as Renilla and firefly luciferase reporters 24 h before IFN treatment. The firefly construct is IFN inducible, whereas the Renilla construct is constitutively expressed. Dose responses of IFNs were performed in quadruplicates. Mean and s.d. are shown. ( d ) HepG2 cells were treated with IFNλ4-S70 or IFNλ4-P70 for 24 h and subsequently infected with EMCV. Cell survival was analysed using the conversion of MTT to formazan in living cells by measurement of the A 600 . Data are presented as a percentage of a non-infected cell control. Error bars depict s.d. of 10 replicates. Full size image rs117648444 A is an independent predictor of HCV clearance If the active IFNλ4 protein is the causative agent responsible for the poor HCV clearance in patients, then one would expect the P70S substitution ( rs117648444 ) to influence the ability of patients to clear HCV. Thus, we evaluated the role of the rs117648444 A (IFNλ4-S70, MAF=0.11) and rs368234815 ΔG (expressing IFNλ4, MAF=0.35) polymorphisms in HCV clearance in a cohort of 574 chronically infected patients who underwent pegIFNα/ribavirin treatment, as well as in 122 patients with spontaneous clearance ( Table 1 ; Supplementary Tables 2 and 3 ). We analysed the independent contribution of each polymorphism, by including both of them in the same logistic regression model. As expected, rs368234815 ΔG was associated with a lower SVR rate (odds ratio (OR)=0.23, 95% confidence interval (CI) 0.15–0.35, P =1.5E-11, dominant mode of inheritance), while rs117648444 A (IFNλ4-S70) was associated with a higher SVR rate (OR=1.66, 95% CI 1.08–2.55, P =0.02). Thus, both rs117648444 A and rs368234815 ΔG are independent predictors of treatment-induced HCV clearance. A similar trend was observed for spontaneous clearance (OR=0.21, 95% CI 0.13–0.34, P =4.4E-10 for rs368234815 ΔG ; OR=1.63, 95% CI 0.88–3.02, P =0.12 for rs117648444 A ; Table 1 ). Table 1 Association between IFNL4 rs368234815 and rs117648444 polymorphisms and spontaneous and treatment-induced HCV clearance. Full size table Stratification of patients according to IFNλ4 functionality A haplotype analysis was performed to understand the co-inheritance pattern of rs368234815 and rs117648444 , which would help to clarify the role of the activity of IFNλ4 in HCV clearance. This analysis showed that 95% of the chromosomes are composed of three main haplotypes: TT G (65%), which is predicted not to produce IFNλ4, ΔG G (22%), which is predicted to produce the IFNλ4-P70 variant, and ΔG A, which is predicted to express the IFNλ4-S70 variant (11%; Supplementary Table 4 ). The frequency distribution in our study population is in accordance with previously published data [15] , [18] . The fourth haplotype TT A, which does not express IFNλ4, was found in only 0.5% of the chromosomes, and is grouped with the TT G haplotype in the subsequent analyses. 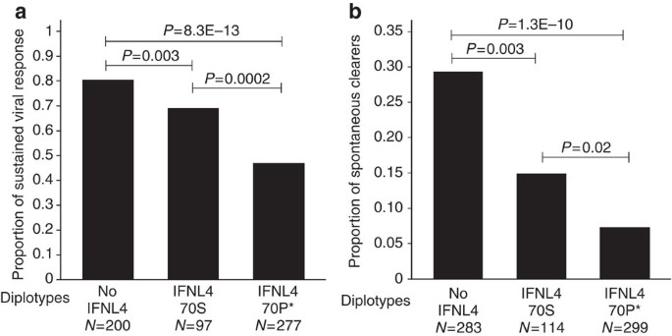Figure 2: Association ofIFNL4 rs368234815andrs117648444polymorphisms and their diplotypes with treatment-induced and spontaneous HCV clearance. Patients were divided into three groups based on their diplotype: those predicted not to produce IFNλ4, those predicted to produce IFNλ4-S70 and those predicted to produce IFNλ4-P70. The latter group included 29 patients (*) with a diplotype encoding both IFNλ4-P70 and IFNλ4-S70. Data represent the proportion of patients infected with all HCV genotypes, who achieved (a) sustained virological response after treatment with pegIFNα/ribavirin or (b) spontaneous clearance.Pvalues were obtained by logistic regression.N=number of patients in a given group. The ΔG G haplotype (IFNλ4-P70, R 2 =0.74) was in linkage disequilibrium (LD) with the SNP rs8099917 , which emerged as the top hit for spontaneous or treatment-induced HCV clearance in three out of four initial hepatitis C genome-wide association studies (GWAS; Table 2 ). Table 2 Linkage disequilibrium between different IFNL4 polymorphisms. 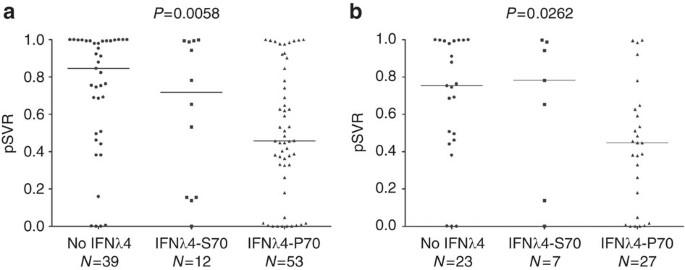Figure 3: Association ofIFNL4genotype with ISG expression in liver biopsies. Overall ISG expression in liver biopsies was assessed with the 4-gene classifier calculating the probability of a sustained virological response for pegIFNα/ribavirin treatments. A high pSVR corresponds to low overall ISGs expression in the liver and vice versa. The biopsies were grouped according to theirIFNL4diplotype as indicated. Shown are results including (a) all HCV genotypes or (b) HCV genotype 1 only. Statistical analysis with Kruskal–Wallis revealed significant overall differences of the median pSVR of the three groups for all genotypes and for genotype 1 only, withP=0.0058 andP=0.026, respectively. Between groups, only the groups ‘no IFNλ4’ and ‘IFNλ4 P70’ were significantly different from each other (Dunn’s multiple comparison test).N=number of samples per group. Full size table The haplotypic combinations produced eight diplotypes ( Table 3 ), which can be classified into three main functional groups according to their ability to produce IFNλ4-P70 or IFNλ4-S70. The first group consists of patients not producing IFNλ4 ( N =283). The second group contains diplotypes that exclusively code for IFNλ4-S70 ( N =114). The third group consists of those that give rise to the fully functional IFNλ4-P70 ( N =299). This group is composed of 270 samples with the TT G/ΔG G and the ΔG G/ΔG G diplotype producing only the IFNλ4-P70 variant, and 29 samples with the ΔG A/ΔG G diplotype producing both variants of IFNλ4. Table 3 IFNL4 haplotype combination and associated clearance phenotypes. Full size table IFNλ4-S70 associates with a better clearance rate of HCV We analysed the response to treatment in patients producing IFNλ4-S70 alone and those producing IFNλ4-P70 alone grouped with IFNL4-P70/S70 compared with those not producing IFNλ4. Patients not producing IFNλ4 had an overall SVR rate of 81% after treatment with pegIFNα/ribavirin compared with only 47% among those who produced the IFNλ4-P70 or P70/S70 variants (OR=0.21, 95% CI 0.14–0.33, P =8.3E−13; Table 1 ; Fig. 2a ). We then excluded patients not producing IFNλ4 to specifically assess the role of the P70S substitution. Interestingly, patients who produced exclusively the IFNλ4-S70 had a much higher response rate (69%) compared with those producing the IFNλ4-P70 or P70/S70 variants (OR=2.52, 95% CI 1.55–4.13, P =0.0002). This clearly shows that the chance of clearing the virus is highest in the group of patients not expressing IFNλ4, slightly lower in those expressing the impaired IFNλ4-S70 variant and the worst in those expressing the fully active IFNλ4-P70 form. The differences in SVR rates between all three groups were significant. This agrees well with the biochemical data, which show that IFNλ4-S70 has an impaired but still clearly measurable activity. These associations were still significant in a multivariate model after adjustment for relevant covariates ( Table 1 ). The association was similar, although less significant, when the analysis was restricted to patients infected with HCV genotype 1 ( Supplementary Table 5 ). Figure 2: Association of IFNL4 rs368234815 and rs117648444 polymorphisms and their diplotypes with treatment-induced and spontaneous HCV clearance. Patients were divided into three groups based on their diplotype: those predicted not to produce IFNλ4, those predicted to produce IFNλ4-S70 and those predicted to produce IFNλ4-P70. The latter group included 29 patients (*) with a diplotype encoding both IFNλ4-P70 and IFNλ4-S70. Data represent the proportion of patients infected with all HCV genotypes, who achieved ( a ) sustained virological response after treatment with pegIFNα/ribavirin or ( b ) spontaneous clearance. P values were obtained by logistic regression. N =number of patients in a given group. Full size image Roughly, a quarter of all HCV-infected individuals spontaneously clear the HCV infection, mainly during the acute phase of the infection by mounting an efficient immune response to the virus [21] . We investigated whether the level of IFNλ4 activity was associated with the spontaneous clearance. Similarly to what was observed for the treatment-induced clearance, the proportion of patients with spontaneous clearance was 29% among patients unable to produce IFNλ4, 7% among those producing the IFNλ4-P70 or P70/S70 variants and 15% among those producing exclusively IFNλ4-S70 ( Table 1 ; Fig. 2b ). IFNλ4-P70 is associated with high ISG expression We have previously shown that the quantification of the expression of four ISGs ( IFI27 , ISG15 , RSAD2 and HTATIP2 ) in liver biopsy samples allows one to predict the response to pegIFNα/ribavirin treatment [10] . This 4-gene classifier was obtained through a multivariate analysis using decision tree ensembles in the form of a random forest classifier and is expressed as the probability of obtaining a sustained virological response (pSVR). The pSVR value contains the collective information from the four genes measured and is inversely correlated with ISG expression in the liver [10] . In the present work, the 4-gene classifier was used as a surrogate marker for the overall ISG expression in 104 liver biopsies from patients with chronic hepatitis C. The biopsies were then genotyped for the IFNλ4 variants and classified into the three groups corresponding to the genomic analysis described above. In an analysis including all viral genotypes, the median pSVR was 85% in group 1 (no IFNλ4, N =39), 72% in group 2 (functionally defective IFNλ4-S70, N =12) and 46% in group 3 (fully functional IFNλ4-P70, N =53). The difference between groups 1 and 3, but not between 1 and 2, was statistically significant ( Fig. 3a ). The results did not change when the analysis was restricted to patients infected with HCV genotype 1 ( Fig. 3b ). Thus, there is a clear correlation between the activity of the IFNλ4 protein and the hepatic ISG expression level. Figure 3: Association of IFNL4 genotype with ISG expression in liver biopsies. Overall ISG expression in liver biopsies was assessed with the 4-gene classifier calculating the probability of a sustained virological response for pegIFNα/ribavirin treatments. A high pSVR corresponds to low overall ISGs expression in the liver and vice versa. The biopsies were grouped according to their IFNL4 diplotype as indicated. Shown are results including ( a ) all HCV genotypes or ( b ) HCV genotype 1 only. Statistical analysis with Kruskal–Wallis revealed significant overall differences of the median pSVR of the three groups for all genotypes and for genotype 1 only, with P =0.0058 and P =0.026, respectively. Between groups, only the groups ‘no IFNλ4’ and ‘IFNλ4 P70’ were significantly different from each other (Dunn’s multiple comparison test). N =number of samples per group. Full size image Because IFNλ4-P70, but not the functionally defective IFNλ4-S70, is associated with a strong induction of ISG expression (and therefore a low pSVR), we conclude that IFNλ4 is the major component of the molecular mechanisms responsible for hepatic ISG expression in patients with HCV infections. Sustained signalling through the IFNλ receptor can inhibit subsequent responses to type I IFN through the induction of the USP18 protein [22] , [23] . Therefore, prolonged IFNλ signalling caused by the IFNλ4 protein is obviously inhibitory to subsequent treatment with pegIFNα/ribavirin. Interestingly, previous work has observed an association between both SNP rs12979860 (ref. 14 ) (situated in the IFNL4 intronic region) and rs368234815 (ref. 13 ) (the ΔG allele determining IFNλ4 expression) and the rate of spontaneous clearance of HCV. We observed a clear correlation between the activity of IFNλ4 and the spontaneous clearance rate. Patients producing the impaired IFNλ4-S70 had a 15% chance of spontaneous clearance compared with a 7% clearance rate among patient coding for the active IFNλ4-P70 variant. Among patients homozygous for the rs368234815 TT allele (major allele, causing a IFNL4 frame shift mutation), the clearance rate was increased to 29%. As the majority of spontaneous clearance occurs during the acute phase of HCV infection, the IFNλ4 protein must influence the early phase of an HCV infection in a way that is favouring development of a chronic infection and thus impairing spontaneous clearance. We speculate that the IFNλ4 protein can influence adaptive immunity, which is established during the acute phase, and that this is a long-lasting influence. Our data link the active form of IFNλ4 (IFNλ4-P70) to high ISG expression and thus to low level of viral replication, which somewhat counterintuitively leads to poor treatment response. We suggest that IFNλ4-P70-driven ISG expression causes lower level of viral replication, which in turn leads to an inefficient adaptive immune response, and that this is the base of poor HCV clearance. This is supported by a recent study showing an association between the rs368234815 ΔG allele (IFNλ4 expression) and activity level of T cells [24] . Furthermore, our findings are supported by a recent paper, showing that patients carrying the IFNλ4-S70-coding allele exhibit a faster decline in HCV RNA levels at week 4 of treatment [25] . Combining rs368234815 and rs117648444 polymorphisms, it is possible to stratify patients into three groups, with the highest cure rates in patients not producing IFNλ4, intermediate cure rates among those producing the IFNλ4-S70 variant and the lowest cure rates among those producing the IFNλ4-P70 variant. Furthermore, there is an excellent agreement between the predicted response rate (pSVR) obtained by measuring ISG expression in liver biopsies and the experientially observed SVR, once patients are stratified according to the three groups defined above. In our cohort, 26% of the patients being able to express IFNλ4 harbour only the IFNλ4-S70 variant, and thus have a prognosis that is almost as good as those not producing IFNλ4. Thus, by combining both polymorphisms, it is possible to substantially improve the accuracy of the predicted response rate before treatment. In addition, we can clarify a discrepancy that has puzzled the field. The rs368234815 polymorphism that determines the ability to express IFNλ4 is not in LD with rs8099917 , which was found as a good SVR predictor in three out of four of the initial GWAS studies [3] , [4] , [5] , [6] . This was unexpected and did initially argue against the IFNλ4 protein as the causative agent; however, it is now clear that the minor allele of rs8099917 specifically tags the haplotype producing the IFNλ4-P70 variant, which we have shown to be associated with the poorest clearance rates. One may argue that the use of genetic markers may become obsolete with the advent of direct-acting antiviral agents (DAAs), due to their high cure rates [26] , [27] , [28] . Nevertheless, the role of IFNL3/IFNL4 polymorphisms has been convincingly demonstrated in the first generation DAA treatment regimes. The SOUND-C2 trial assessing the combination of faldaprevir and deleobuvir with or without ribavirin showed a significantly higher SVR rates for patients homozygous for the favourable allele of rs12979860 (CC), clearly demonstrating a role for IFNL genotype in IFN-free DAA treatment regimens [29] . Thus, in mechanistic term, the role of the IFNL genotype is not restricted to IFN-based therapies, but do influence DAA-based treatments. However, recent development in DAA combination therapies using drugs with a substantially improved potency has pushed SVR above 90% for all patients, regardless of their IFNL genotype. With cure rates, this high knowledge of the genotype will have little impact on patients’ choices of treatment. However, there are several clinical as well as scientific reasons to pursue a deeper understanding of how IFNL genotype impact viral clearance. Several recent studies show that rs368234815 influences the response kinetics to DAA [28] , [30] ; however, the role of rs117648444 in DAA treatment has not yet been investigated. This suggests that patients not expressing IFNλ4 can receive a shortened DAA treatment and possibly also reduced doses. There will be both obvious benefits for patients and substantial cost reduction by a targeted shortening of therapy in patients with favourable IFNL genotype. Our study clearly shows that the decision should be based on a dual genotyping of rs117648444 and rs368234815 . The expression of active IFNλ4 influences both IFN-based and IFN-free treatment of chronic HCV infections, as well as strongly influences the spontaneous clearance rate. These observations point towards a fundamental role of active IFNλ4 in facilitating and maintaining a chronic HCV infection. A recent study showed that rs368234815 also influenced susceptibility to cytomegalovirus retinitis among HIV-infected patients [31] , suggesting that the IFNλ4 protein might play detrimental role in several different chronic viral infections. Thus, we believe that the activity of IFNλ4 could play an important role in multiple chronic viral infections by a mechanism similar to that observed in hepatitis C. Protein expression and purification BL21 (DE3) E. coli cells transformed with the plasmids were grown at 37 °C in Luria Bertani medium containing 100 μg ml −1 ampicillin and 100 μl antifoam A concentrate (Sigma‐Aldrich, catalogue number A5633) under continuous shaking until an OD 600 of 0.8–1. Protein expression was induced by adding 1 mM isopropyl‐β‐D‐thiogalactopyranoside and incubating for another 4 h at 37 °C. Refolding and purification were performed as previously described [32] . The His-tag was removed by the tobacco etch virus (TEV) protease cleavage after the refolding was completed. The TEV was removed during the subsequent cation exchange chromatography using a HiTrap SP FF column. The TEV cleavage was omitted for IFNλ3. It is worth noting that the yield of IFNλ4 protein is low with 1–2 mg of purified protein from 12 l E. coli culture. We did not note any consistent differences in the expression levels between IFNλ4-P70 and IFNλ-S70. Plasmids The IFNλ4-S70 constructs were generated by site‐directed mutagenesis using PfuUltra II Fusion HS DNA polymerase according to the manufacturer’s instructions (Agilent). For the mammalian cell expression, pEF2-IFNλ4-S70-FLAG was generated on pEF2-IFNλ4-P70-FLAG template using forward 5′-CCGCGGAGAATCCCTCCTGGGGC-3′ and reverse 5′-GCCCCAGGAGGGATTCTCCGCGG-3′ primers. For the expression in E. coli , pET15b-IFNλ4-S70 was generated on pET15b-IFNλ4-P70 construct using forward 5′-GCTGCTCGGACGAGGCGAATCACGACGCGGACG-3′ and reverse 5′-CGTCCGCGTCGTGATTCGCCTCGTCCGAGCAGC-3′ primers. The following PCR programme was used: (1) 95 °C for 30 s; (2) 16 cycles of 95 °C for 30 s, 65 °C for 1 min and 72 °C for 4 min; and (3) 72 °C for 10 min. Cell culture Unless otherwise stated, all cells were grown in Dulbecco’s modified Eagle’s medium (DMEM), which was supplemented with 10% fetal bovine serum, 100 U ml −1 penicillin and 100 μg ml −1 streptomycin. Cells were purchased from the German Collection of Microorganisms and Cell Cultures, DSMZ (HepG2 DSMZ-No. : ACC-180; HEK293 DSMZ-No. : ACC-305). Activity assay in HEK293 cells HEK293 cells were seeded at a density of 7.5 × 10 4 cells per well in a 48‐well plate and left to rest for 24 h. After 24 h, the cells were transfected with the pEF2 plasmid encoding IFNλR1, firefly luciferase under the control of the Mx1 promoter [33] and Renilla luciferase under the control of the β ‐ actin promoter. Eighteen hours post-transfection, cells were induced in quadruplicates with eight dilutions of IFNλ4-P70 and IFNλ4-S70 in the concentration range covering 0.006–100 ng ml −1 for 24 h. After 24 h, the cells were washed with PBS and lysed with Passive Lysis Buffer (Promega). The lysates were spun down at 10,000 g for 2 min at 4 °C, and the cleared lysates were used for the measurement of luciferase activity (Dual‐Luciferase Reporter Assay System, Promega). EC 50 , efficacy and exponential slope values were estimated in GraphPad prism version 5.04 by fitting a sigmoidal equation to the plot. The equation used for fitting was: firefly/Renilla ratio=baseline+(efficacy−baseline)/ ( 1 + 10 ((logEC 50 − X ) × Slope ) . Values for baseline were restrained to zero. Real‐time quantitative PCR HepG2 cells were seeded at a density of 2 × 10 5 cells per well in 12‐well plates, and after 24 h, fresh media were added with the indicated IFNs in quadruplicates. After 4 h of incubation, cells were lysed and RNA was purified using an extraction kit (Omega) according to the manufacturer’s instructions. Complementary DNA synthesis was performed with 1 μg RNA using RevertAid reverse transcriptase and random hexamer primer according to the manufacturer’s instructions (Thermo Scientific). The cDNA obtained from cells was quantified by real-time quantitative PCR using SYBR Green I (Roche) on Roche LightCycler 480 II. The following primers were used: GAPDH , forward 5′-CGACCACTTTGTCAAGCTCA-3′ and reverse 5′-GGTGGTCCAGGGGTCTTACT-3′; IFIT1 , forward 5′-CCTCCTTGGGTTCGTCTACA-3′ and reverse 5′-GGCTGATATCTGGGTGCCTA-3′; and MX1 , forward 5′-ACCTACAGCTGGCTCCTGAA-3′ and reverse 5′-CGGCTAACGGATAAGCAGAG-3′. The cycling parameters were: 95 °C for 10 min followed by 45 cycles of 95 °C for 10 s, 60 °C for 20 s and 72 °C for 12 s. The crossing points of the amplification curves were determined using the second derivate method on the Roche 480 LightCycler software 1.5 (Roche). The level of mRNA was normalized against the GAPDH mRNA content. The mean of the quadruplicates of the untreated control was used to calculate the fold induction for the other samples. Antiviral assay HepG2 cells were seeded at a concentration of 1.8 × 10 4 cells per well in 96-well plates and incubated with 20 dilutions of IFNλ4-P70 or IFNλ4-S70 in the concentration range covering 0.008–200 ng ml −1 for 24 h. The cells were then infected with EMCV (VR-129B strain) at a multiplicity of infection of 0.45. After 24 h, MTT (3-(4,5-dimethylthiazol-2-yl)-2,5-diphenyl tetrazolium bromide; Sigma Aldrich) was added at a concentration of 0.8 mg ml −1 in DMEM, and the cells were incubated for additional 4 h. The cells were dissolved in dimethyl sulfoxide (Sigma-Aldrich). MTT conversion was determined by measurement of the A 600 . Measured absorptions in the IFN wells (Abs) were normalized as a percent of the cell control (CC) with the virus control (VC) subtracted, using the following equation: normalized cell survival (NCS)=(Abs−VC/(CC−VC)) × 100 to allow activity comparisons between plates. EC 50 , efficacy and exponential slope values were estimated as described in the section entitled ‘Activity assay in HEK293 cells’. Liver biopsies Liver biopsies from patients ( n =104) were obtained in the outpatient clinic of the Division of Gastroenterology and Hepatology, University Hospital Basel, Switzerland. Parts of the biopsy material that were not needed for routine histopathology were used for research purposes after obtaining written informed consent. The use of biopsy material for this project was approved by the Ethikkommission Nordwest- und Zentralschweiz, Basel, Switzerland. Serum HCV RNA was quantified using the Cobas AmpliPrep/COBAS TaqMan HCV Test and the Cobas Amplicor Monitor from Roche Molecular Systems (Basel, Switzerland). Total RNA and genomic DNA were isolated from liver biopsies using Trizol reagent (Invitrogen, Basel, Switzerland) and DNeasy Blood & Tissue Kit (Qiagen, Hombrechtikon, Switzerland) according to the manufacturer’s instructions. A fragment of 850 base pair covering rs368234815 and rs117648444 was amplified with the Expand High Fidelity PCR System (Roche) using forward 5′-ACTGTGTGTGCTGTGCCTTC-3′ and reverse 5′-GGACGAGAGGGCGTTAGAG-3′ primers. The product was purified on a column using NucleoSpin Gel and PCR clean-up (Macherey-Nagel AG, Oensingen, Switzerland) according to the manufacturer’s instructions and then sequenced (Microsynth AG, Balgach, Switzerland). pSVR was calculated using the 4-classifier genes as described previously [10] . Statistical analysis was performed using Prism6 (GraphPad software. La Jolla, CA, USA). Genetic association study Samples from patients with written informed consent for genetic studies and available DNA were collected from the Swiss Hepatitis C Cohort Study (SCCS), a multicenter study of HCV-infected patients enroled at eight major Swiss hospitals and their local affiliated centres, as described previously [16] , [34] , and from the Liver Unit of the Casa Sollievo della Sofferenza, San Giovanni Rotondo, Italy. The study was approved by the Ethics Committee of each SCCS center (Ethikkommission beider Basel EKBB (Basel), Ethikkommission des Kantons St Gallen (St Gallen), Comité intercantonal d'éthique (Neuchâtel), Comité d'éthique du département de Médecine (Geneva), Department Innere Medizin Ethisches Komitee (Zurich), Commission d'éthique de la recherche clinique (Lausanne), Comitato etico cantonale (Lugano)) and by the Ethical committee of ‘Casa Sollievo della Sofferenza’. The study included Caucasian patients with spontaneous HCV clearance (defined as presence of anti-HCV antibodies but undetectable HCV RNA without previous antiviral treatment) and those who had chronic infection with HCV genotypes 1, 2, 3 or 4 and were assessable for response to therapy with pegIFNα and ribavirin, that is, who received >80% of the recommended dose of each drug. Polymorphisms in the IFNL3/4 region ( rs12979860, rs368234815, rs117648444 and rs8099917) were extracted from a GWAS-generated data set [4] or genotyped by TaqMan (Applied Biosystems, Rotkreuz, Switzerland) or by the Competitive Allele Specific PCR (KASP) system (LGC Genomics, Herts, UK; http://www.lgcgenomics.com/kaspchallenge ). Haplotypes were inferred using PHASE software, version 2.1 (University of Washington, available through Express Licensing Program, Seattle, WA, USA; http://stephenslab.uchicago.edu/software.html ). Statistical analyses were performed using Stata (version 13.1, StataCorp LP, College Station, TX, USA). LD was assessed using the programs PWLD implemented in Stata. The association of polymorphisms with response to treatment and spontaneous clearance was performed by univariate and multivariate logistic regression. The multivariate models for spontaneous clearance are adjusted for age, sex and HCV risk. The multivariate models for response to treatment are adjusted age, sex, fibrosis stage and viral genotype. How to cite this article: Terczyńska-Dyla, E. et al. Reduced IFNλ4 activity is associated with improved HCV clearance and reduced expression of interferon-stimulated genes. Nat. Commun. 5:5699 doi: 10.1038/ncomms6699 (2014).